Respiratory transmission of an avian H3N8 influenza virus isolated from a harbour seal The ongoing human H7N9 influenza infections highlight the threat of emerging avian influenza viruses. In 2011, an avian H3N8 influenza virus isolated from moribund New England harbour seals was shown to have naturally acquired mutations known to increase the transmissibility of highly pathogenic H5N1 influenza viruses. To elucidate the potential human health threat, here we evaluate a panel of avian H3N8 viruses and find that the harbour seal virus displays increased affinity for mammalian receptors, transmits via respiratory droplets in ferrets and replicates in human lung cells. Analysis of a panel of human sera for H3N8 neutralizing antibodies suggests that there is no population-wide immunity to these viruses. The prevalence of H3N8 viruses in birds and multiple mammalian species including recent isolations from pigs and evidence that it was a past human pandemic virus make the need for surveillance and risk analysis of these viruses of public health importance. Beginning in September 2011, over 160 young harbour seals ( Phoca vitulina) were found moribund or dead along the New England coast. After ruling out common causes of death, an avian influenza subtype H3N8 virus was identified [1] . Influenza H3N8 viruses are one of the most commonly found subtypes in wild birds [2] and are associated with mild to no disease in infected birds. Unlike many avian subtypes, H3N8 viruses have a broad host range, have been associated with ongoing outbreaks in dogs [3] and horses [4] and have been isolated from pigs [5] , donkeys [6] and now seals [1] . This suggests that these predominantly avian viruses easily cross species barriers and establish lineages in mammals. Influenza viruses (H3N3, H4N5, H4N6 and H7N7) have previously been isolated from seals with respiratory symptoms, and H4N5 and H7N7 have been associated with large-scale mortality events [7] , [8] , [9] , [10] . During one of the H7N7 seal outbreaks, four persons in close contact with diseased seals developed conjunctivitis demonstrating that direct transmission to humans can occur [10] . The full extent of H3N8 virus exposure in harbour seals is unknown. In previous mortality events, up to 20% of the local seal population died and it was estimated that between 3 and 5% of the total harbour seal population in the northeast perished [8] . Depending on location, timing and species tested, serological surveys in the United States and Canada have reported between 0 and 26% of the seals had prior exposure to influenza viruses. Genomic characterization of the A/harbour seal/New Hampshire/179629/2011(H3N8) virus revealed that it was closely related to avian influenza viruses from wild birds and exhibited no reassortment with mammalian influenza viruses [1] . In spite of this relatedness to wild bird viruses, and unlike previous seal influenza viruses [7] , [8] , [9] , [10] , the 2011 seal virus contained a number of mutations associated with mammalian pathogenicity [1] including Q222, G224 and T315 mutations in the haemagglutinin (HA) protein that were shown to confer highly pathogenic avian H5N1 viruses the ability to transmit via respiratory droplets [11] , [12] . Further, the virus acquired a substitution in the PB2 gene known to increase pathogenicity in mice [13] . Combined, these studies suggest that the seal H3N8 virus, although wholly derived from birds, may have the ability to cause enhanced disease and potentially transmit among mammals. Here, to test this possibility, a panel of avian H3N8 influenza viruses is evaluated for replication in vitro , and pathogenicity and transmission in vivo. The panel includes avian H3N8 strains A/mallard/Alberta/274/1979 (mallard/274), A/mallard/Alberta/50/1979 (mallard/50), A/mallard/Alberta/551/2009 (mallard/551), A/ruddy duck/Illinois/3471/2009 (ruddy duck), A/long-tailed duck/Maine/295/2011 (long-tailed duck), an isolate that was collected from New England sea birds during the same time frame as the seal outbreak and the A/harbour seal/New Hampshire/179629/2011 (harbour seal) strain. The well-studied [7] , [14] , [15] , [16] , [17] reference H3N8 virus [18] , A/duck/Ukraine/1/1963 (duck/Ukraine), with known receptor-binding affinity [19] , [20] , [21] is used as a control for in vitro and in vivo experiments. Seal and related avian H3N8 viruses form a distinct subclade Phylogenetic analysis of the H3 HA genes showed that these viruses cluster into distinct clades. The duck/Ukraine virus clusters with Eurasian avian viruses, which are hypothesized to be the progenitors of historical and currently circulating H3 viruses in humans [14] , [16] , [22] , [23] . In contrast, the seal, ruddy duck ( Oxyura jamaicensis ) and long-tailed duck ( Clangula hyemalis ) viruses clustered with more contemporary North American avian viruses isolated from migratory birds in North and Central America ( Fig. 1a ), while the mallard ( Anas platyrhynchos ) viruses cluster within an older subclade of North American wild bird isolates, demonstrating that there are clear genetic differences amongst the avian H3 viruses used in these studies including four distinct amino acid changes (I58M, S141N, V159L and V238I) in the head region of the HA within the subclade containing the seal virus ( Fig. 1b ). 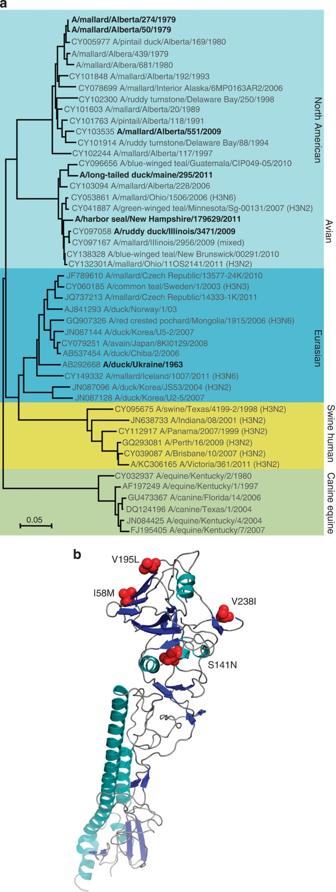Figure 1: Genetic relationship amongst H3 hemagglutinin genes. (a) Phylogenetic tree for H3 HA gene. The genetic relationship of the H3N8 HA genes was determined by aligning nucleotide sequences, and the tree is drawn to scale with branch lengths in the same units as those of the evolutionary distances used to infer the phylogenetic tree. (b) Amino acid changes associated with viruses in the harbour seal clade. Four amino acid changes were observed between harbour seal associated viruses and viruses in the second North American avian subclade. All four amino acids were located in the head domain of the HA protein. Figure 1: Genetic relationship amongst H3 hemagglutinin genes. ( a ) Phylogenetic tree for H3 HA gene. The genetic relationship of the H3N8 HA genes was determined by aligning nucleotide sequences, and the tree is drawn to scale with branch lengths in the same units as those of the evolutionary distances used to infer the phylogenetic tree. ( b ) Amino acid changes associated with viruses in the harbour seal clade. Four amino acid changes were observed between harbour seal associated viruses and viruses in the second North American avian subclade. All four amino acids were located in the head domain of the HA protein. Full size image Seal H3N8 virus has increased affinity for α2,6 sialic acids Given that these amino acid changes surround the receptor-binding domain, solid-phase glycan-binding assays were performed and revealed that the seal virus had greater binding affinity for mammalian-type (α2,6) sialic acids similar to the human A/California/04/2009 (CA/09, pdmH1N1) and A/Perth/16/2009 (seasonal human H3N2) viruses as compared with the other avian viruses that had greater affinity for avian-type (α2,3) linkages similar to duck/Ukraine control virus [19] , [20] ( Fig. 2 ). Ligand concentration calculation ( K d ) based on absorbance from binding assays showed that the human and seal viruses bound to α2,6 sialic acids in the sub-μg ml −1 range, while the non-seal clade avian viruses bound α2,3 sialic acids in a similar range ( Supplementary Table 1 ). In contrast, the seal clade, long-tailed duck and ruddy duck viruses bound with similar affinity to both α2,6 and α2,3 sialic acids although more quantitative analyses are required on a larger subset of viruses to determine if this is a unique feature of this clade. In summation, these findings expand on previous work demonstrating that the harbour seal virus binds to both α2,6 and α2,3 ligands [1] . 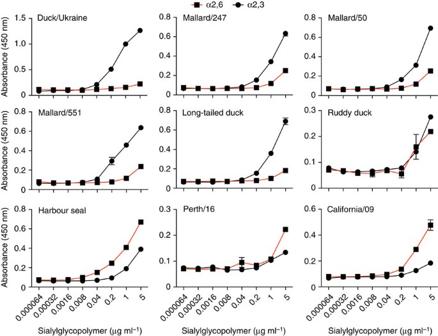Figure 2: Sialic acid binding affinities of the different viruses. Viruses associated with the harbour seal clade had increased binding to α2,6 sialic acids suggesting increased mammalian binding efficiency. Data are representative of two experiments with three replicates per virus. Error bars represent the s.e. of the mean. Figure 2: Sialic acid binding affinities of the different viruses. Viruses associated with the harbour seal clade had increased binding to α2,6 sialic acids suggesting increased mammalian binding efficiency. Data are representative of two experiments with three replicates per virus. Error bars represent the s.e. of the mean. Full size image Seal virus has efficient respiratory droplet transmission On the basis of the differences in receptor specificity among the avian H3N8 viruses, ferrets were intranasally inoculated with 10 6 50% tissue culture infectious dose (TCID 50 ) units of the duck/Ukraine, mallard/50, mallard/551, ruddy duck, long-tailed duck and seal viruses. One day post inoculation (d.p.i. ), naïve ferrets were either placed with the infected group (direct contact transmission) or, in the case of the seal virus, housed in cages adjacent to the donor ferrets, separated by grills, to allow unobstructed airflow while preventing direct contact (respiratory droplet transmission). Animals were monitored for disease signs through 14 d.p.i., nasal washes collected every 2 d.p.i. to assess viral shed and seroconversion determined at 14 d.p.i. Although 100% of the inoculated animals shed virus between 2 and 6 d.p.i. and seroconverted ( Fig. 3 ), only the strains genetically related to the seal virus were transmitted to the direct contact animals ( Fig. 3d–f ). Interestingly, the long-tailed duck virus only transmitted to two out of three direct contacts, while the ruddy duck virus transmitted to 100% of contacts. Most importantly, the seal virus transmitted by respiratory droplet to two out of three contacts between days 5 and 7 post exposure ( Fig. 3g ). While no overt clinical signs of disease were observed in animals following infection, ferrets inoculated with the harbour seal virus were observed sneezing from 2 to 4 d.p.i., and one of the aerosol contact animals was observed sneezing on day 6 pi. Viruses recovered from the aerosol contact ferrets had an A134T change within the HA, which has been shown to alter the receptor-binding specificity of H5N1 viruses from α2,3 to α2,6 sialic acid linkages [24] , [25] . 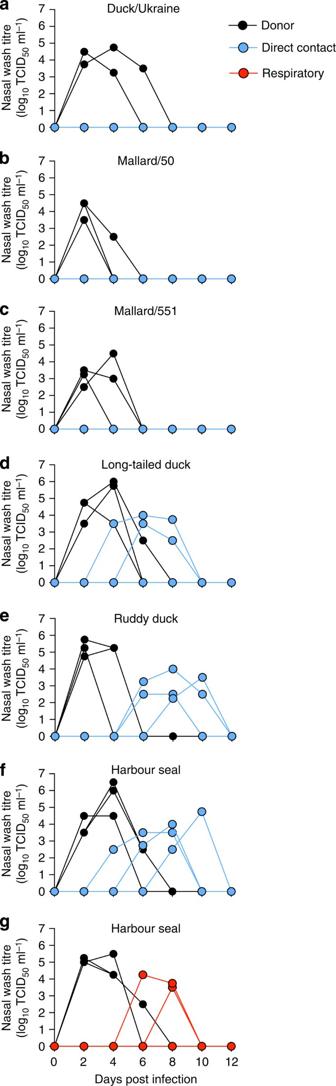Figure 3: Transmission of H3N8 viruses. (a–g) Ferrets (n=3 per group/experiment,n=2 for control avian virus) were inoculated with 106units of H3N8 influenza virus (black lines). Twenty-four hours later, naïve ferrets (n=2–3) were either placed in direct contact with the infected group (blue lines) or housed in separate cages (respiratory transmission, red lines) and nasal washes were collected on the indicated d.p.i. for virus quantification. Lines represent individual animals. Data are representative of three separate experiments for seal H3N8 and two separate experiments for other viruses. Figure 3: Transmission of H3N8 viruses. ( a – g ) Ferrets ( n =3 per group/experiment, n =2 for control avian virus) were inoculated with 10 6 units of H3N8 influenza virus (black lines). Twenty-four hours later, naïve ferrets ( n =2–3) were either placed in direct contact with the infected group (blue lines) or housed in separate cages (respiratory transmission, red lines) and nasal washes were collected on the indicated d.p.i. for virus quantification. Lines represent individual animals. Data are representative of three separate experiments for seal H3N8 and two separate experiments for other viruses. Full size image Seal and related H3N8 viruses replicate efficiently in vitro To further characterize the virulence and pathogenicity of the avian and mammalian H3N8 viruses, replication was evaluated in cell culture and mice. Briefly, Madin–Darby Canine Kidney (MDCK), human lung adenocarcinoma A549 cells and differentiated normal human bronchial epithelial (NHBE) cells cultured at an air–liquid interface were infected at a multiplicity of infection of 0.01–0.03 and viral titres determined at indicated times post infection by TCID 50 analysis on MDCK cells [26] . Viruses associated with the seal clade replicated faster at early time points in all cell types studied ( Fig. 4a–c ). The seal and closely related avian viruses had increased titres early in infection and replicated to higher titres overall compared with the non-seal clade and control avian viruses in A549 cells ( Fig. 4b ). Although not as striking, a similar trend was seen with NHBE cells with increased viral titres at 24 h post infection (h.p.i., Fig. 4c ). Overall, these studies demonstrate that the avian viruses genetically related to the seal virus can productively replicate in human cells. 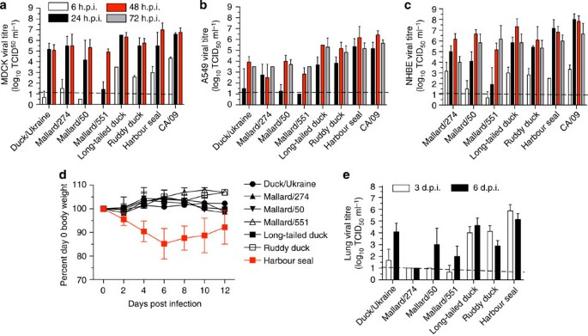Figure 4: Replicative capacity of H3N8 virusesin vitroandin vivo. To evaluate the replication of the H3N8 virusesin vitro, MDCK (a) human lung A549 (b) or primary NHBE cells grown in an air–liquid interface (c) were infected at an multiplicity of infection of 0.01–0.03 (NHBE) and cell culture supernatants collected at 6, 24, 48 and 72 h.p.i. Viral titres were determined by TCID50analysis in triplicate. Data are representative of at least two experiments. Error bars represent the s.e. of the mean. To evaluate the pathogenicity and transmissibility of avian and mammalian H3N8 viruses 6–8-week-old BALB/c mice (n=10/group/experiment) were i.n. infected with 105TCID50units of the indicated viruses and weight loss (d) was monitored for 12 d.p.i. (e) At 3 and 6 d.p.i., lungs were collected from three mice per group and viral titres were determined in homogenates by TCID50analysis. Error bars represent the s.e. of the mean. Data are representative of two experiments. Figure 4: Replicative capacity of H3N8 viruses in vitro and in vivo . To evaluate the replication of the H3N8 viruses in vitro , MDCK ( a ) human lung A549 ( b ) or primary NHBE cells grown in an air–liquid interface ( c ) were infected at an multiplicity of infection of 0.01–0.03 (NHBE) and cell culture supernatants collected at 6, 24, 48 and 72 h.p.i. Viral titres were determined by TCID 50 analysis in triplicate. Data are representative of at least two experiments. Error bars represent the s.e. of the mean. To evaluate the pathogenicity and transmissibility of avian and mammalian H3N8 viruses 6–8-week-old BALB/c mice ( n =10/group/experiment) were i.n. infected with 10 5 TCID 50 units of the indicated viruses and weight loss ( d ) was monitored for 12 d.p.i. ( e ) At 3 and 6 d.p.i., lungs were collected from three mice per group and viral titres were determined in homogenates by TCID 50 analysis. Error bars represent the s.e. of the mean. Data are representative of two experiments. Full size image Seal and related H3N8 viruses replicate efficiently in mice Finally, to monitor pathogenicity, Balb/c mice were intranasally inoculated with each virus at a dose of 10 5 TCID 50 units, weight loss was monitored for 12 d.p.i. and viral titres determined on days 3 and 6 p.i. ( Fig. 4d,e ). As opposed to the non-seal clade and duck/Ukraine virus, all of the viruses genetically similar to the seal virus replicated well in the lungs of infected mice by 3 d.p.i. ( Fig. 4e ), although only the seal virus caused significant weight loss and clinical scores compared with uninfected controls ( Fig. 4d ). Seasonal vaccination fails to protect against seal virus To test whether seasonal vaccination would confer protection against the harbour seal H3N8 virus, haemagglutination inhibition (HI) studies were performed with baseline and post-vaccination sera from 102 individuals collected between 2009 and 2011 (ref. 27 ). While all individuals readily seroconverted against the seasonal H3 virus (A/Brisbane/10/2007 or A/Perth/16/2009 depending on vaccination year), only one individual displayed any pre-existing antibodies against the harbour seal virus (1:30) and this titre did not increase following vaccination. Microneutralization assays against harbour seal H3N8 were negative (data not shown). Further, convalescent sera from ferrets infected with the harbour seal virus showed no cross reaction with human H3N2 vaccine strains in HI assays ( Supplementary Table 2 ). Given the genetic distance between the human and harbour seal H3 viruses ( Fig. 1a ), the lack of cross-protection was not surprising. Although these were only a small panel of human samples, these studies suggest a lack of population-wide immunity to the avian H3N8 viruses. In summary, our work has demonstrated that the seal virus is unique amongst the avian H3N8 viruses tested having enhanced α2,6 receptor binding, increased morbidity in mice and efficient respiratory droplet transmission in ferrets. Numerous avian influenza subtypes including H1, H2, H3, H6, H7 and H9 viruses have been assessed for mammalian pathogenicity and transmission [28] , [29] , [30] , [31] , [32] , [33] , [34] , [35] , [36] . However, only a very few, specifically the H1, H2, H9 and H7 subtypes [28] , [29] , [30] , [31] , [34] , [35] , [36] , transmit via limited direct contact and only the newly emergent H7N9 viruses transmit by respiratory droplet [31] , [34] ( Supplementary Table 3 ). Although only the seal virus transmitted via respiratory droplets, the other avian viruses within this clade efficiently transmitted via contact. This may be a unique feature of this clade worthy of further studies. The transmissibility of the seal H3N8 virus coupled with the apparent lack of immunity makes these strains a concern. Indeed, implication of the H3N8 virus as a past human pandemic virus [37] , the recent isolation of this subtype in pigs [5] and the potential acquisition of mammalian adaptation phenotypes make the need for surveillance and risk analysis of these viruses of public health importance. Further studies are needed to determine the molecular determinants associated with respiratory droplet transmission of the seal virus and determine how readily the other avian viruses within this clade can gain these changes. Indeed, the efficient respiratory droplet transmission and replication of this clade of H3N8 virus indicate that mammalian-transmissible, avian influenza viruses may already exist in nature. Viruses All of the viruses were propagated in the allantoic cavity of 10-day-old specific pathogen-free embryonated chicken eggs at 37 °C. Allantoic fluid was collected, cleared by centrifugation and stored at −80 °C (refs 38 , 39 ). Sequencing and sequence analysis For virus segments not available from Genebank, the complete coding region of all genomic segments were directly sequenced and phylogenetically analysed. Amplicons were purified and sequenced by the Sanger method in the Hartwell Center at St. Jude Children’s Research Hospital. Sequences were aligned using ClustalW and Bioedit [40] , [41] . The eight gene segments were phylogenetically analysed on the basis of their nucleotide sequences. Phylogenetic analyses were carried out using MEGA version 5.05, with the neighbor-joining method, Kimura two-parameter model [42] . Bootstrap values (1,000 replications and >60) are indicated on the tree. Viruses were clustered on the basis of nucleotides, and only dominant clusters were used to infer phylogenetic relationships. Receptor-binding assays Receptor affinity was determined using a solid-phase direct virus binding assay as previously described [19] , [25] . Briefly, influenza viruses were bound to fetuin-coated plates at 4 °C overnight. Biotinylated glycans (α2,3'SL or α2,6'SL, Glycotech Coorporation, Gaithersburg, MD) were added to influenza-coated plates at varying dilutions and incubated for a further 4 h. Glycan binding was analysed using HRP-conjugated streptavidin (Invitrogen, Carlsbad, CA) followed by TMB substrate (Sigma, St Louis, MO) and plates were read at 450 nm on a Synergy 2 multi-mode microplate reader (BioTek Instruments, Winooski, VT). Kd was determined by Linear Regression analysis using GraphPad Prism 5 software. Cells and culture media MDCK cells were cultured in Eagle’s minimum essential medium (MediaTech, Manassas, VA) supplemented with 2 mM glutamine and 10% fetal bovine sera (Gemini BioProducts, West Sacramento, CA) and grown at 37 °C under 5% CO 2 . A549 cells were cultured in Dulbecco’s minimum essential medium (DMEM, Lonza, Walkersville, MD) supplemented with 4.5 g l −1 glutamine and 10% fetal bovine serum and grown at 37 °C under 5% CO 2 . Well-differentiated (transepithelial resistance greater than 1,000), primary NHBE were purchased from MatTek Corp (Ashland, MA), maintained by daily washes with 0.9% sodium chloride solution (Sigma, St Louis, MO) and incubated at the air–liquid interface at 37 °C under 5% CO 2 . The basal surface was in contact with AIR 100 growth media (MatTek Corp) with complete growth medium being replaced every 24 h. In vitro infections A549 and MDCK cells were infected with a multiplicity of infection of 0.01 for 1 h at 37 °C. Cells were washed three times to remove unbound virus and infected cells were cultured in appropriate media containing 0.075% bovine serum albumin and 1 μg ml −1 TPCK-treated trypsin. Aliquots of culture supernatants were collected at 6, 24, 48 and 72 h.p.i. and immediately stored at −80 °C for the determination of virus titres. For infection of NHBE cells, basal medium was removed and replaced with DMEM. The apical surface was washed twice and incubated with fresh, serum-free DMEM containing virus for 2 h at 37 °C after which both apical and basal medium was removed and fresh growth medium was added to the basal chamber as described [26] . At 6, 24, 48 and 72 h.p.i., DMEM was added to the apical surface and incubated for 30 min at 37 °C. This media was collected and stored at −80 °C for determination of virus titres. Animal experiments All animal experiments were approved by the St. Jude Children’s Research Hospital Animal Care and Use Committee. Six to 8-week-old female BALB/c mice (Jackson Laboratory, Bar Harbour, ME; n =16 mice/group) were lightly anaesthetized with isofluorane and intranasally inoculated with PBS or 10 5 TCID 50 units of virus in 25 μl PBS. Mice were monitored daily for clinical signs of infection and weighed every 48 h.p.i. [43] . At days 3 and 6 p.i., three control and infected mice were euthanized and lungs were collected and homogenized in 1 ml PBS. Viral titres determined by TCID 50 analysis [26] , [38] . Data are representative of two separate experiments. For transmission studies, 9–15-week-old male ferrets ( n =3, Triple F Farms, Sayre, PA) were inoculated intranasally with 10 6 TCID 50 units in 1 ml PBS. Twenty-four hours later, naïve ferrets ( n =3 per each group) were either placed in direct contact with the infected group or housed in separate cages. Body weight and temperature were assessed every 48 h and the ferrets were monitored for the following clinical signs: anorexia, sneezing, nasal discharge and lethargy. Nasal washes were collected at every 2 days p.i. for viral titration and sera collected at 14 d.p.i. for HI analysis as described [44] . Experiments were repeated three times for harbour seal virus and two times for the other viruses for a total n =6–9 ferrets per group. Human serology Human sera were collected as part of ongoing prospective observational study carried out at the University of North Carolina Family Medicine Center between 2009 and 2011. All procedures were approved by the Biomedical Institutional Review Board at the University of North Carolina [27] . Haemagglutination inhibition (HI) assay was conducted to determine the level of antibodies in sera. Briefly, sera were treated with receptor-destroying enzyme (RDE; Denka Seiken, Tokyo, Japan) overnight, followed by inactivation at 56 °C for 1 h, and a final dilution to 1:10 with PBS. Receptor-destroying enzyme-treated sera were then incubated in duplicate with A/harbour seal/New Hampshire/179629/2011 (H3N8) virus for 15 min at room temperature. After 30 min incubation at 4 °C with 0.5% turkey red blood cells, HAI titre was determined by the reciprocal dilution of the last well. Positive and negative controls as well as back titrations of virus were included on each individual plate. To determine cross-reactivity against human H3N2 viruses, convalescent sera were collected from A/harbour seal/New Hampshire/179629/2011-infected animals and HAI assays were conducted as described above. How to cite this article: Karlsson, E. A. et al . Respiratory transmission of an avian H3N8 influenza virus isolated from a harbour seal. Nat. Commun. 5:4791 doi: 10.1038/ncomms5791 (2014). Accession codes: Sequencing data has been deposited in the GenBank database under accession codes KJ467564 , KJ467565 , KJ467566 , KJ467567 , KJ467568 , KJ467569 , KJ467570 and KJ467571 .